Histone modifications and lamin A regulate chromatin protein dynamics in early embryonic stem cell differentiation Embryonic stem cells are characterized by unique epigenetic features including decondensed chromatin and hyperdynamic association of chromatin proteins with chromatin. Here we investigate the potential mechanisms that regulate chromatin plasticity in embryonic stem cells. Using epigenetic drugs and mutant embryonic stem cells lacking various chromatin proteins, we find that histone acetylation, G9a-mediated histone H3 lysine 9 (H3K9) methylation and lamin A expression, all affect chromatin protein dynamics. Histone acetylation controls, almost exclusively, euchromatin protein dynamics; lamin A expression regulates heterochromatin protein dynamics, and G9a regulates both euchromatin and heterochromatin protein dynamics. In contrast, we find that DNA methylation and nucleosome repeat length have little or no effect on chromatin-binding protein dynamics in embryonic stem cells. Altered chromatin dynamics associates with perturbed embryonic stem cell differentiation. Together, these data provide mechanistic insights into the epigenetic pathways that are responsible for chromatin plasticity in embryonic stem cells, and indicate that the genome's epigenetic state modulates chromatin plasticity and differentiation potential of embryonic stem cells. Chromatin and nuclear architecture in embryonic stem cells (ESCs) have several unique properties when compared with somatic or differentiated cells. Undifferentiated ESCs possess fewer condensed heterochromatin foci, which are larger and more dispersed than those of early differentiating cells [1] and a less structured nuclear lamina [2] , which is devoid of lamin A [3] (LMNA). LMNA is directly associated with chromatin [4] , [5] and may thus confer nuclear rigidity and chromatin stability in differentiated cells. In undifferentiated ESCs, the organization of chromatin seems to be more homogeneous, and the DNA is distributed more evenly throughout the nucleus as compared with somatic cells or neuronal progenitor cells (NPCs) derived from ESCs by in vitro differentiation [6] . Moreover, chromatin in ESCs is characterized by hyperdynamic binding of architectural chromatin proteins including heterochromatin protein 1 (HP1), histone H1 and core histones [7] . Significantly, restriction of this dynamic state, using a tightly bound H1 mutant (H1cc), which we previously generated, interferes with ESC self-renewal and differentiation potential [7] , suggesting that the hyperdynamic state of chromatin proteins is functionally important for the stem cell state. ESCs are also distinguished by a unique epigenetic landscape. Developmentally regulated genes are enriched with histone marks of both active (H3K4me) and inactive (H3K27me) chromatin [8] , [9] , [10] , rendering them primed for the onset of a transcriptional program that will lead to differentiation [11] , [12] . In addition, in undifferentiated ESCs, the levels of acetylated histones are generally increased, while the levels of heterochromatin-associated histone modifications, such as histone H3 tri-methylated on lysine 9 (H3K9me3), are generally reduced [2] , [13] . Finally, silent chromatin marked by H3K9me2 accumulates in the form of large blocks during ESC differentiation [14] . Taken together, these data underline the importance of chromatin and its epigenetic landscape for the maintenance of both cellular pluripotency and the differentiated state, and call for studying the mechanisms regulating chromatin plasticity in ESCs. To investigate the molecular mechanisms underlying the hyperdynamic nature of chromatin in ESCs, in this study we focussed on the dynamic mobility of histone H1 (H1–GFP fusion protein), which, as it has an intermediate level of dynamics between the highly dynamic HP1 proteins and the stably bound core histones [7] , [15] , is an excellent indicator of chromatin plasticity in ESCs [7] . We analysed H1 dynamics and differentiation potential in several mutant ESCs that lack various chromatin-related proteins, including Suv39h1/2 −/− , G9a −/− , Lmna −/− , Dnmt1 −/− , Dnmt3a/3b −/− , Dnmt1/3a/3b −/− and H1c/d/e −/− , as well as following treatments with DNA de-methylating agents, histone acetyltrasnferase inhibitor and histone deacetylase inhibitors (HDACi). We found that the epigenetic state of the genome, particularly histone acetylation and histone methylation, as well as LMNA expression, affect chromatin plasticity and the differentiation potential of ESCs. Specifically, increased histone acetylation is associated with increased plasticity and protein dynamics on euchromatin, while H3K9 methylation regulates both euchromatin and heterochromatin protein dynamics and ectopic expression of LMNA exclusively restricts heterochromatin protein dynamics. In contrast, DNA methylation and nucleosome repeat length have little effect on chromatin protein dynamics. These results provide mechanistic insights into the regulation of chromatin plasticity in ESCs and pave the way for the manipulation of pluripotency by chromatin-related mechanisms. Histone acetylation increases H1 dynamics in euchromatin Previously, we reported that both linker and core histones display hyperdynamic association with chromatin in undifferentiated ESCs [7] . To investigate the potential mechanisms leading to this property, we tested different cells and treatments using H1–GFP fusion protein as an indicator for chromatin plasticity. Undifferentiated ESCs exhibit elevated levels of acetylated histones compared with differentiated cells [6] , [7] , [16] , hence we investigated whether these higher acetylation levels contribute to the hyperdynamic nature of chromatin-associated proteins in ESCs [7] . To this end, we examined the effects of HDACi on chromatin protein dynamics in somatic mouse embryonic fibroblasts (MEFs) and in mouse ESCs. We treated H1–GFP-expressing cells with low levels (0.5 mM) of the HDACi valproic acid (VPA) for 24 h before subjecting them to fluorescence recovery After Photobleaching (FRAP) [7] , analysing euchromatin and heterochromatin separately [15] . We detected a significant increase in the dynamic association of H1–GFP with euchromatin in MEFs ( Fig. 1a ), but not with heterochromatin ( Fig. 1b ). Similar behaviour was observed in undifferentiated R1 ESCs, with a significant increase in euchromatin ( Fig. 1c ) but not in heterochromatin ( Fig. 1d ), although initial levels of H1 kinetics were higher in ESCs and the relative increase was lower (compare Fig. 1a with Fig. 1c ). Similar results were observed for a 4-h treatment with either VPA or the HDACi trichostatin A (TSA) ( Fig. 1e–l ). Increased acetylation levels were verified by western blotting ( Fig. 2a ). To test whether changes in H1 dynamics mark a general chromatin hyperdynamics pattern, we examined chromatin association dynamics of HP1 and of HMGN1 in ESCs—the dynamic binding of these two proteins to chromatin has been studied in detail [7] , [17] ; once again, similar results were observed ( Supplementary Fig. S1 ), ruling out the possibility that the effect is due to acetylation or other modifications of H1 itself. Increased dynamics was more significant in euchromatin than heterochromatin ( Fig. 1 ), suggesting differences in the accessibility to HDACs or in the nucleosomes' basic interaction with chromatin proteins. Regardless, increased histone acetylation correlates with increased chromatin protein dynamics in euchromatin in both somatic cells and ESCs. 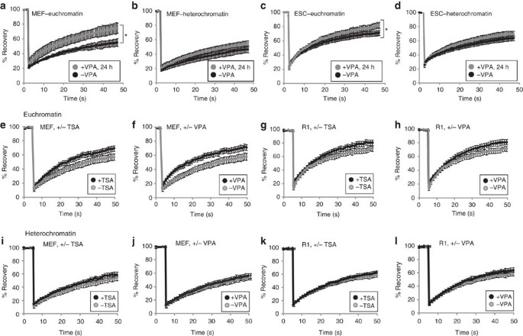Figure 1: Increased histone acetylation increases H1 dynamics. (a–d) FRAP analysis (± s.d.) of H1e–GFP in euchromatin (a,c) and heterochromatin (b,d) in MEFs (a,b) and in R1 mouse ESCs (c,d) treated (grey) or untreated (black) with the HDAC inhibitor VPA for 24 h. Changes for euchromatin are significant (a,P<0.005;c,P<0.01;d,P>0.05, 2-tailedt-test). (e,f) FRAP analysis of H1e–GFP in euchromatin of MEFs treated (black) or untreated (grey) with TSA (e) or VPA (f) for 4 h. Changes are significant (P<0.005 in both cases, 2-tailedt-test). (g,h) FRAP analysis of H1e–GFP in euchromatin of mouse ESCs treated (black) or untreated (grey) with TSA (g) or VPA (h) for 4 h. Changes are significant (P<0.05 in both cases, 2-tailedt-test). (i,j) FRAP analysis of H1e–GFP in heterochromatin of MEFs treated (black) or untreated (grey) with TSA (i) or VPA (j) for 4 h. (k,l) FRAP analysis of H1e–GFP in heterochromatin of ESCs treated (black) or untreated (grey) with TSA (k) or VPA (l) for 4 h. Values are from at least 2 independent experiments, at least 20 cells each. Error bars represent s.d. Figure 1: Increased histone acetylation increases H1 dynamics. ( a – d ) FRAP analysis (± s.d.) of H1e–GFP in euchromatin ( a , c ) and heterochromatin ( b , d ) in MEFs ( a , b ) and in R1 mouse ESCs ( c , d ) treated (grey) or untreated (black) with the HDAC inhibitor VPA for 24 h. Changes for euchromatin are significant ( a , P <0.005; c , P <0.01; d , P >0.05, 2-tailed t -test). ( e , f ) FRAP analysis of H1e–GFP in euchromatin of MEFs treated (black) or untreated (grey) with TSA ( e ) or VPA ( f ) for 4 h. Changes are significant ( P <0.005 in both cases, 2-tailed t -test). ( g , h ) FRAP analysis of H1e–GFP in euchromatin of mouse ESCs treated (black) or untreated (grey) with TSA ( g ) or VPA ( h ) for 4 h. Changes are significant ( P <0.05 in both cases, 2-tailed t -test). ( i , j ) FRAP analysis of H1e–GFP in heterochromatin of MEFs treated (black) or untreated (grey) with TSA ( i ) or VPA ( j ) for 4 h. ( k,l ) FRAP analysis of H1e–GFP in heterochromatin of ESCs treated (black) or untreated (grey) with TSA ( k ) or VPA ( l ) for 4 h. Values are from at least 2 independent experiments, at least 20 cells each. Error bars represent s.d. 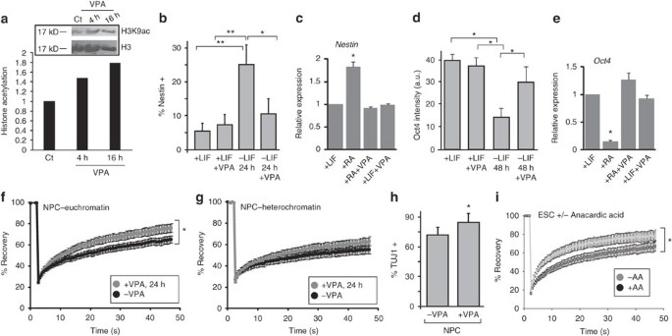Figure 2: Increased histone acetylation affects pluripotency and differentiation. (a) Western blot (inset) and densitometric quantification of histone acetylation levels following 4 and 16 h of VPA treatment. Unmodified histone H3 was used for normalization. (b) In the presence of LIF, ~5% of the ESC colonies display nestin-positive cells. When LIF is removed, ~25% of the cells become nestin-positive after 24 h (P=3×10−8, 2-tailedt-test), but this number drops to ~10% when the cells are also treated with VPA (P<0.05, 2-tailedt-test).yAxis denotes the % of nestin-positive colonies. (c) Quantitative real-time RT–PCR analyses ofnestinexpression in R1 ESCs treated or untreated with RA for 48 h in the absence or presence of VPA. (d) Over 95% of undifferentiated ESCs were Oct4-positive.Oct4levels were significantly reduced 48 h after LIF withdrawal but largely restored when also treated with VPA (P<0.05, 2-tailedt-test). At least 100 cells were analysed in 2 independent experiments.yAxis denotes fluorescence intensity. (e) Quantitative real-time RT–PCR analyses of Oct4 expression in R1 ESCs treated or untreated with RA for 48 h in the absence or presence of VPA. (f,g) FRAP analysis of H1e–GFP in 7-days NPCs differentiated from ESCs treated (grey) or untreated (black) with VPA in both euchromatin (f) and heterochromatin (g). Changes for euchromatin are significant (P<0.05, 2-tailedt-test). (h) VPA treatment increases TUJ1 positive cells from ~74 to ~84% (P<0.05, 2-tailedt-test). At least 100 cells were analysed in 2 independent experiments. (i) FRAP analysis of H1e–GFP in ESCs treated (black) or untreated (grey) with AA for 1 h. Changes are significant (P<0.05, 2-tailedt-test). In panelsa–eandh, values are from 2–3 biological replicates; in panelsf–gandi, values are from at least 2 independent experiments, at least 20 cells each. Error bars represent s.d. Full size image Figure 2: Increased histone acetylation affects pluripotency and differentiation. ( a ) Western blot (inset) and densitometric quantification of histone acetylation levels following 4 and 16 h of VPA treatment. Unmodified histone H3 was used for normalization. ( b ) In the presence of LIF, ~5% of the ESC colonies display nestin-positive cells. When LIF is removed, ~25% of the cells become nestin-positive after 24 h ( P =3×10 −8 , 2-tailed t -test), but this number drops to ~10% when the cells are also treated with VPA ( P <0.05, 2-tailed t -test). y Axis denotes the % of nestin-positive colonies. ( c ) Quantitative real-time RT–PCR analyses of nestin expression in R1 ESCs treated or untreated with RA for 48 h in the absence or presence of VPA. ( d ) Over 95% of undifferentiated ESCs were Oct4-positive. Oct4 levels were significantly reduced 48 h after LIF withdrawal but largely restored when also treated with VPA ( P <0.05, 2-tailed t -test). At least 100 cells were analysed in 2 independent experiments. y Axis denotes fluorescence intensity. ( e ) Quantitative real-time RT–PCR analyses of Oct4 expression in R1 ESCs treated or untreated with RA for 48 h in the absence or presence of VPA. ( f , g ) FRAP analysis of H1e–GFP in 7-days NPCs differentiated from ESCs treated (grey) or untreated (black) with VPA in both euchromatin ( f ) and heterochromatin ( g ). Changes for euchromatin are significant ( P <0.05, 2-tailed t -test). ( h ) VPA treatment increases TUJ1 positive cells from ~74 to ~84% ( P <0.05, 2-tailed t -test). At least 100 cells were analysed in 2 independent experiments. ( i ) FRAP analysis of H1e–GFP in ESCs treated (black) or untreated (grey) with AA for 1 h. Changes are significant ( P <0.05, 2-tailed t -test). In panels a – e and h , values are from 2–3 biological replicates; in panels f – g and i , values are from at least 2 independent experiments, at least 20 cells each. Error bars represent s.d. Full size image Next, we examined how HDACi affect the differentiation propensity of ESCs. Interestingly, E14 ESCs treated with VPA for 24 h demonstrate a reduced propensity to differentiate in the absence of leukaemia inhibitory factor (LIF). When induced to differentiate by LIF withdrawal, the number of the neuroectodermal marker nestin-positive E14 ESC colonies increased from ~5 to ~25%, but when treated with VPA, 90% of the colonies remained nestin-negative ( Fig. 2b ). To confirm these results at the population level and with a different differentiation method, we performed qRT–PCR on RNA extracted from undifferentiated ESCs±retinoic acid (RA) and ±VPA for 48 h and measured messenger RNA levels of nestin. RA alone increased nestin levels by almost twofold, but this increase was prevented by VPA ( Fig. 2c ). VPA alone did not significantly change nestin mRNA levels ( Fig. 2c ). We also analysed the expression levels of additional mesodermal ( Brachyury ) and endodermal ( GATA4 ) differentiation markers. RA significantly reduced Brachyury and significantly increased GATA4 , but these trends were reversed in the presence of VPA ( Supplementary Fig. S2 ). We also analysed levels of pluripotency markers. After 48 h of LIF withdrawal, Oct4 intensity in ESCs was reduced to 35% of control levels ( Fig. 2d ). However, in the presence of VPA, Oct4 levels were restored to 76% of original levels ( Fig. 2d ). This was confirmed independently with RA for 48 h, in the absence or presence of VPA. Once again, low levels of VPA reduced RA-induced differentiation ( Fig. 2e ). These results suggest that HDACi-induced histone hyperacetylation in ESCs supports the undifferentiated state. However, HDACi do not affect the expression levels of pluripotency genes in ESCs [18] , [19] , suggesting an indirect effect, possibly through altering global chromatin structure to a more open state [20] . Together, these data show that elevated histone acetylation may be an underlying mechanism regulating chromatin hyperdynamics in undifferentiated ESCs and suggest that persistent hyperdynamics may have an inhibitory effect on differentiation, implying a potential functional link between chromatin dynamics and differentiation capacity. We next examined the effect of HDACi on ESC-derived NPCs, which have lower chromatin protein dynamics than undifferentiated ESCs [7] . Indeed, increased H1–GFP dynamics was observed in NPCs treated with VPA for 24 h ( Fig. 2f,g ). Interestingly, whereas HDACi largely maintain ESCs in an undifferentiated state ( Fig. 2b–e ; Supplementary Fig. S2 ), VPA-treatment of NPCs slightly increased neuronal differentiation rather than halting it, as judged by the percentage of β-Tubulin-III (TUJ1)-positive cells after 24 h (from 73.5±8.5% in the untreated NPCs to 84.4±11.0% in the VPA-treated NPCs; Fig. 2h ). This result is consistent with a previous report, which demonstrated that, in hippocampal neural progenitor cells, VPA prevented gliogenesis and promoted neurogenesis [21] . Finally, we analysed the effects of a histone acetyltransferase inhibitor anacardic acid (AA) on H1–GFP dynamics in ESCs. As expected, the dynamic association of H1–GFP with chromatin was significantly reduced in ESCs treated for 1 h with 50 μM of AA ( Fig. 2i ). We repeated these experiments in differentiating ESCs after 4 days of RA treatment and found a similar restriction of H1–GFP dynamics in both AA-treated and non-treated cells, as previously observed [7] . Taken together, these results show that histone acetylation regulates chromatin protein mobility in euchromatin, and apparently maintains ESCs undifferentiated while facilitating neuronal differentiation of NPCs. H3K9 methylation affects H1 dynamics in ESCs Relatively low H3K9 methylation levels are a hallmark of chromatin in undifferentiated ESCs [7] , [13] , [14] and thus a promising candidate for restricting chromatin plasticity during ESC differentiation. We tested previously characterized mutant ESCs that lack either G9a (ref. 22 ) or Suv39h1/2 (ref. 23 ), the H3K9 histone methyltransferases. As ESCs gain H3K9 methylation following differentiation, we compared between mutant and WT undifferentiated ESCs and differentiating NPCs. We detected no difference in the dynamic association of H1–GFP with chromatin in Suv39h1/2 mutant cells; however, in G9a −/− ESCs, H1–GFP dynamics were not restricted following differentiation by RA treatment for 4 days, as observed in WT ESCs [7] ( Fig. 3a–d ). In G9a −/− ESCs with G9a re-introduced (G9a-Add-WT) [24] , normal kinetics were observed with reduced H1–GFP dynamics following differentiation ( Fig. 3e,f ). In contrast, when a mutant G9a lacking catalytic activity was re-introduced into G9a −/− ESCs (G9a-Add-Mut) [24] , the Null phenotype was observed ( Fig. 3g,h ), suggesting that G9a catalytic activity is required to restrict chromatin protein dynamics during ESC differentiation. Because G9a mutants can still form heterodimers with GLP and bind chromatin [24] , chromatin binding is not sufficient to mediate restriction of chromatin dynamics. 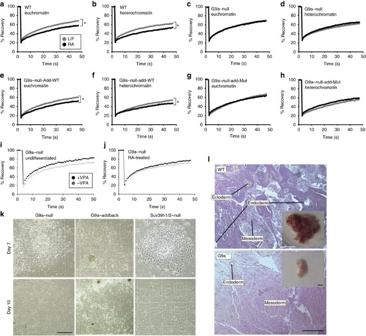Figure 3: H3K9 methylation affects H1 dynamics and differentiation. (a,b) H1e–GFP FRAP analysis in euchromatin (a) and heterochromatin (b) of WT ESCs, undifferentiated (LIF, grey) or differentiated with retinoic acid for 4 days (RA, black). Changes are significant (P<0.01, 2-tailedt-test). (c,d) H1e–GFP FRAP analysis in euchromatin (c) and heterochromatin (d) of G9a−/−ESCs, undifferentiated (grey) or differentiated with RA for 4 days (black). No restriction of H1 dynamics is observed following differentiation. (e,f) H1e–GFP FRAP analysis in euchromatin (e) and heterochromatin (f) of G9a−/−ESCs in which WT G9a was added-back (G9a-Null-add-WT), undifferentiated (grey) or differentiated with RA for 4 days (black). Changes are significant (P<0.05, 2-tailedt-test). (g,h) H1e–GFP FRAP analysis in euchromatin (g) and heterochromatin (h) of G9a−/−ESCs in which a mutant form of G9a lacking catalytic activity was added-back (G9a-Null-add-Mut), undifferentiated (grey) or differentiated with RA for 4 days (black). No restriction of chromatin protein dynamics is observed following differentiation. (i,j) H1e–GFP FRAP analysis in G9a−/−ESCs, undifferentiated (i) and differentiated for 4 days with RA (j), treated (black) or untreated (grey) with 0.5 mM VPA for 24 h. In both cases, changes are significant (P<0.005, 2-tailedt-test). (k) Neuronal differentiation of G9a−/−, G9a-addback and Suv39h1/2−/−ESCs. All cells reach the NPC stage at day 7 (top) but the G9a−/−cells die between day 7 and day 10 while the G9a-addback and the Suv39h1/2−/−cells continue to differentiate normally. Scale bar, 100 μm. (l) Teratoma analysis in SCID mice injected with WT (top) or G9a−/−(bottom) ESCs. WT ESCs displayed normal differentiation with apparent endoderm, mesoderm and ectoderm. However, teratomas made from G9a−/−ESCs were significantly smaller (inset) and did not show neuroectodermal differentiation. Scale bar, 0.5 mm; inset scale bar, 5 mm. Values are from at least 2 independent experiments, at least 20 cells each. Figure 3: H3K9 methylation affects H1 dynamics and differentiation. ( a , b ) H1e–GFP FRAP analysis in euchromatin ( a ) and heterochromatin ( b ) of WT ESCs, undifferentiated (LIF, grey) or differentiated with retinoic acid for 4 days (RA, black). Changes are significant ( P <0.01, 2-tailed t -test). ( c , d ) H1e–GFP FRAP analysis in euchromatin ( c ) and heterochromatin ( d ) of G9a −/− ESCs, undifferentiated (grey) or differentiated with RA for 4 days (black). No restriction of H1 dynamics is observed following differentiation. ( e , f ) H1e–GFP FRAP analysis in euchromatin ( e ) and heterochromatin ( f ) of G9a −/− ESCs in which WT G9a was added-back (G9a-Null-add-WT), undifferentiated (grey) or differentiated with RA for 4 days (black). Changes are significant ( P <0.05, 2-tailed t -test). ( g , h ) H1e–GFP FRAP analysis in euchromatin ( g ) and heterochromatin ( h ) of G9a −/− ESCs in which a mutant form of G9a lacking catalytic activity was added-back (G9a-Null-add-Mut), undifferentiated (grey) or differentiated with RA for 4 days (black). No restriction of chromatin protein dynamics is observed following differentiation. ( i , j ) H1e–GFP FRAP analysis in G9a −/− ESCs, undifferentiated ( i ) and differentiated for 4 days with RA ( j ), treated (black) or untreated (grey) with 0.5 mM VPA for 24 h. In both cases, changes are significant ( P <0.005, 2-tailed t -test). ( k ) Neuronal differentiation of G9a −/− , G9a-addback and Suv39h1/2 −/− ESCs. All cells reach the NPC stage at day 7 (top) but the G9a −/− cells die between day 7 and day 10 while the G9a-addback and the Suv39h1/2 −/− cells continue to differentiate normally. Scale bar, 100 μm. ( l ) Teratoma analysis in SCID mice injected with WT (top) or G9a −/− (bottom) ESCs. WT ESCs displayed normal differentiation with apparent endoderm, mesoderm and ectoderm. However, teratomas made from G9a −/− ESCs were significantly smaller (inset) and did not show neuroectodermal differentiation. Scale bar, 0.5 mm; inset scale bar, 5 mm. Values are from at least 2 independent experiments, at least 20 cells each. Full size image To test the relationship between histone methylation and acetylation and to ask whether these pathways are linked in terms of chromatin plasticity, we treated G9a −/− ESCs with VPA for 24 h and measured H1–GFP mobility using FRAP. We found that VPA induced hyperdynamic binding of H1–GFP in G9a −/− ESCs ( Fig. 3i ), as we observed in WT ESCs ( Fig. 1 ). We repeated the experiment in G9a −/− ESCs after 4 days of RA-induced differentiation. Once again, we found that VPA increased mobility of H1–GFP, although to a somewhat lesser extent than the undifferentiated ESCs ( Fig. 3j ). These data suggest that the two pathways of histone acetylation and G9a-mediated methylation are not directly linked and that at least some HDACs bind chromatin in the absence of G9a. We tested whether G9a overexpression would have the opposite effect in ESCs. Overexpressing G9a in WT ESCs for 72 h reduced H1–GFP dynamics ( Supplementary Fig. S3 ). When subjected to in vitro neuronal differentiation, the G9a −/− cells failed to differentiate into stage IV and stage V neurons and died shortly before or shortly after they became stage III NPCs ( Fig. 3k ). In contrast, both G9a-addback (G9a-Add-WT) and Suv39h1/2 −/− ESCs differentiated normally ( Fig. 3k ), although Suv39h1/2 −/− ESCs tended to differentiate spontaneously and precociously in the absence of MEFs. As G9a −/− ESCs failed to generate mature neurons, we tested their differentiation potential in vivo by injecting G9a −/− ESCs into severe combined immunodeficient (SCID) mice and examining the teratomas 21 days later. We found mostly undifferentiated mesoderm and some residual endoderm but very little evidence of neural ectoderm ( Fig. 3l ). This suggests that G9a might be essential not only for proper heterochromatin formation during ESC differentiation, but also for proper differentiation and/or pluripotency of ESCs. Considering the possibility that pluripotency factors directly regulate G9a, we examined ChIP-seq data of pluripotency factors [26] at the G9a locus, but found no association with the G9a promoter. Also, overexpression of pluripotency factors in ESCs [27] did not alter G9a expression levels, and the level and distribution of both H3K9 histone methyltransferases did not change significantly during early ESC differentiation [6] , [28] , [29] . Finally, the levels of pluripotency genes in ESCs remained unaltered in the absence of G9a (ref. 30 ). We conclude that G9a is not directly bound or regulated by pluripotency factors in ESCs. Taken together, these data suggest that increased H3K9 methylation in differentiating ESCs restricts chromatin protein dynamics and that G9a is required for proper differentiation of ESCs. Lamin A partially restricts heterochromatin H1 dynamics We hypothesized that LMNA may be involved in the restriction of chromatin dynamics following ESC differentiation based on several facts. First, LMNA is not detected in undifferentiated ESCs [3] ( Fig. 4a ), and their nuclear lamina, marked by lamin B, appears less structured than in differentiated cells [7] , [31] , [32] , [33] . Moreover, LMNA appears early during differentiation, approximately when chromatin-binding proteins become less mobile [3] . Finally, heterochromatin domains are frequently found at the nuclear periphery and LMNA directly associates with chromatin by binding core histones [4] , [5] . We therefore tested the relationship between LMNA expression and chromatin plasticity. 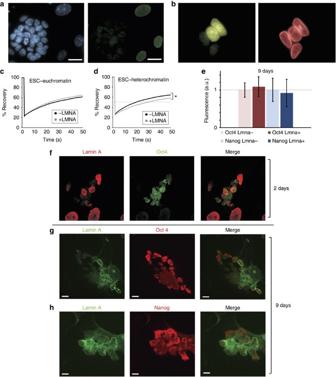Figure 4: LMNA partially restricts H1 dynamics in heterochromatin. (a) Stained with DAPI (blue), an R1 mouse ESC colony is surrounded by three fibroblasts. Fibroblasts stain positive with anti-LMNA antibodies (green); ESCs do not. (b) R1 ESCs were co-transfected with bothLmnaandH1e–GFPat a 10:1 ratio. Anti-LMNA antibodies (red) recognize the exogenously expressed LMNA. Because of the transfection ratio between the two plasmids, all H1e–GFP-positive cells were LMNA-positive. (c,d) H1e–GFP FRAP analysis in R1 ESCs ectopically expressing (grey) or not expressing (black) WT mouse LMNA. No significant changes were observed in euchromatin (c) but changes in heterochromatin (d) are significant (P<0.05, 2-tailedt-test). (e) Quantitative analysis of immunofluorescence levels of Oct4 and Nanog is shown before and after 9 days of ectopic LMNA expression. (f) Forty-eight hours afterLmnatransfection, all R1 ESCs stain positive for Oct4 (green), regardless of whether they stain positive or negative for LMNA (red). The large nuclei are MEFs that served as LMNA-positive controls and Oct4-negative controls. (g,h) Nine days afterLmnatransfection, all R1 ESCs stain positive for Oct4 and Nanog (red), regardless of whether they stain positive or negative for LMNA (green). In all panels, values are from 2–3 biological replicates. Error bars represent s.d. Figure 4: LMNA partially restricts H1 dynamics in heterochromatin. ( a ) Stained with DAPI (blue), an R1 mouse ESC colony is surrounded by three fibroblasts. Fibroblasts stain positive with anti-LMNA antibodies (green); ESCs do not. ( b ) R1 ESCs were co-transfected with both Lmna and H1e–GFP at a 10:1 ratio. Anti-LMNA antibodies (red) recognize the exogenously expressed LMNA. Because of the transfection ratio between the two plasmids, all H1e–GFP-positive cells were LMNA-positive. ( c , d ) H1e–GFP FRAP analysis in R1 ESCs ectopically expressing (grey) or not expressing (black) WT mouse LMNA. No significant changes were observed in euchromatin ( c ) but changes in heterochromatin ( d ) are significant ( P <0.05, 2-tailed t -test). ( e ) Quantitative analysis of immunofluorescence levels of Oct4 and Nanog is shown before and after 9 days of ectopic LMNA expression. ( f ) Forty-eight hours after Lmna transfection, all R1 ESCs stain positive for Oct4 (green), regardless of whether they stain positive or negative for LMNA (red). The large nuclei are MEFs that served as LMNA-positive controls and Oct4-negative controls. ( g , h ) Nine days after Lmna transfection, all R1 ESCs stain positive for Oct4 and Nanog (red), regardless of whether they stain positive or negative for LMNA (green). In all panels, values are from 2–3 biological replicates. Error bars represent s.d. Full size image To test the contribution of LMNA to chromatin dynamics restriction during ESC differentiation, we ectopically expressed LMNA together with H1e–GFP in undifferentiated ESCs and analysed H1e–GFP dynamics. Ectopic LMNA properly localized in the ESC nuclear lamina. This was viewed in live cells expressing Cherry-tagged human- and mouse-LMNA ( Supplementary Fig. S4 ) and in fixed cells that expressed untagged LMNA, detectable by anti-LMNA antibodies ( Fig. 4b ). We used untagged LMNA because anti-LMNA antibodies failed to recognize Cherry-tagged LMNA. Lamin B staining revealed the less structured nuclear lamina in undifferentiated as opposed to differentiated ESCs [2] . H1e–GFP FRAP experiments were performed in ESCs with or without co-expression of LMNA ( Fig. 4b ). When comparing H1e–GFP dynamics in cells co-expressing LMNA with cells transfected only with H1e–GFP, we found a slight reduction in chromatin protein dynamics ( Supplementary Fig. S4e ). We repeated the LMNA and H1e–GFP co-transfection experiments and analysed recovery rates in euchromatin and heterochromatin, separately. Whereas H1e–GFP dynamics displayed similar kinetics in euchromatic regions of LMNA-expressing and non-expressing cells ( Fig. 4c ), a significant reduction in H1 mobility was recorded in discrete heterochromatin foci ( Fig. 4d ). Reduced plasticity was not caused by forced differentiation of LMNA-expressing ESCs because they did not alter their pluripotency markers, 2 or 9 days after transfection ( Fig. 4e–h ). These results indicate that ectopic expression of LMNA in ESCs restricts chromatin protein dynamics exclusively in heterochromatin. We next tested whether LMNA is necessary to restrict chromatin protein dynamics during ESC differentiation. We generated Lmna −/− NPCs ( Fig. 5a,b ) and measured H1e–GFP dynamics in heterochromatin and euchromatin, separately. Interestingly, H1 dynamics restriction, characteristic of the NPC stage or earlier [7] ( Fig. 5c ), was significantly, albeit not entirely, abolished in Lmna −/− NPCs ( Fig. 5d ). Additionally, whereas H1 kinetics in heterochromatin are usually slower than in euchromatin [7] , [15] , [34] , [35] ( Fig. 1 ), in Lmna −/− cells, H1 kinetics in heterochromatin were similarly hyperdynamic as in euchromatin ( Supplementary Fig. S4f–g ). This interesting observation reflects the hyperdynamic heterochromatin in Lmna −/− NPCs, suggesting perturbed heterochromatin formation or maintenance in Lmna −/− ESC differentiation. Confirming this notion, nuclear shape in Lmna −/− NPCs was highly irregular ( Figs 5b and 6b,d), and the number of conspicuous heterochromatin foci was dramatically lower than in WT NPCs ( Fig. 5e,f ). Finally, to check how LMNA affects differentiation potential, we stained Lmna −/− NPCs at day 6 for early and late neuronal markers nestin and β-tubulin-III (TUJ1), respectively. Whereas nestin was detected in both WT and Lmna −/− NPCs, β-tubulin-III was only detected in WT NPCs and was completely absent from Lmna −/− NPCs (37% versus 0%, P <0.005, 2-tailed t -test). 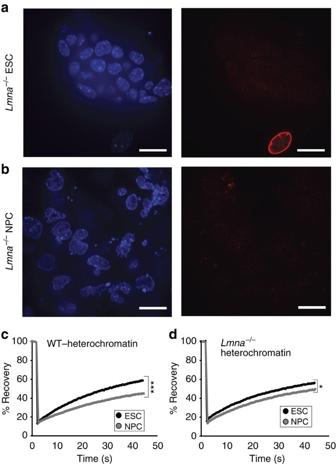Figure 5:Lmna−/−NPCs exhibit reduced heterochromatin restriction. (a,b)Lmna−/−ESCs (a) and NPCs (b) stain negative for LMNA, unlike the fibroblast that expresses LMNA (red). DAPI is shown in blue. Note aberrant nuclear shapes ofLmna−/−NPCs. (c) H1e–GFP FRAP analysis in heterochromatin of undifferentiated R1 ESCs (black) and NPCs (grey). Changes are significant (P<0.001, 2-tailedt-test). (d) H1e–GFP FRAP analysis in heterochromatin of undifferentiatedLmna−/−ESCs (black) and NPCs derived fromLmna−/−ESCs (grey). Changes are significant (P<0.05, 2-tailedt-test). Values are from at least 2 independent experiments, at least 20 cells each. Figure 5: Lmna −/− NPCs exhibit reduced heterochromatin restriction. ( a , b ) Lmna −/− ESCs ( a ) and NPCs ( b ) stain negative for LMNA, unlike the fibroblast that expresses LMNA (red). DAPI is shown in blue. Note aberrant nuclear shapes of Lmna −/− NPCs. ( c ) H1e–GFP FRAP analysis in heterochromatin of undifferentiated R1 ESCs (black) and NPCs (grey). Changes are significant ( P <0.001, 2-tailed t -test). ( d ) H1e–GFP FRAP analysis in heterochromatin of undifferentiated Lmna −/− ESCs (black) and NPCs derived from Lmna −/− ESCs (grey). Changes are significant ( P <0.05, 2-tailed t -test). Values are from at least 2 independent experiments, at least 20 cells each. 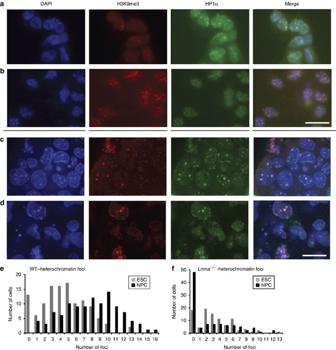Figure 6:Lmna−/−NPCs exhibit abnormal heterochromatin structure. (a,b) DAPI (blue) and immunostaining for heterochromatin markers H3K9me3 (red) and HP1α (green) in WT mouse ESCs (a) and NPCs (b). Scale bar, 20 μm. (c,d) DAPI (blue) and immunostaining for heterochromatin markers H3K9me3 (red) and HP1α (green) inLmna−/−ESCs (c) and inLmna−/−NPCs (d). Scale bar, 20 μm. (e) Distribution of heterochromatin foci number per nucleus in WT ESCs (grey) and NPCs (black). The average number of foci per nucleus increased from 4.5±5.9 in ESCs to 7.9±4.1 in NPCs. (f) Distribution of heterochromatin foci number per nucleus inLmna−/−ESCs (grey) and NPCs (black). The average number of foci per nucleus decreased from 3.3±6.8 in ESCs to 2.6±12.1 in NPCs. At least 100 cells were counted in 2 independent experiments. Full size image Figure 6: Lmna −/− NPCs exhibit abnormal heterochromatin structure. ( a , b ) DAPI (blue) and immunostaining for heterochromatin markers H3K9me3 (red) and HP1α (green) in WT mouse ESCs ( a ) and NPCs ( b ). Scale bar, 20 μm. ( c , d ) DAPI (blue) and immunostaining for heterochromatin markers H3K9me3 (red) and HP1α (green) in Lmna −/− ESCs ( c ) and in Lmna −/− NPCs ( d ). Scale bar, 20 μm. ( e ) Distribution of heterochromatin foci number per nucleus in WT ESCs (grey) and NPCs (black). The average number of foci per nucleus increased from 4.5±5.9 in ESCs to 7.9±4.1 in NPCs. ( f ) Distribution of heterochromatin foci number per nucleus in Lmna −/− ESCs (grey) and NPCs (black). The average number of foci per nucleus decreased from 3.3±6.8 in ESCs to 2.6±12.1 in NPCs. At least 100 cells were counted in 2 independent experiments. Full size image These observations did not recur in Lmna −/− MEFs derived from Lmna −/− mice [36] . Comparing H1e–GFP dynamic association with chromatin in WT versus Lmna −/− MEFs, we detected no significant differences in either euchromatin or heterochromatin regions ( Supplementary Fig. S5 ). Lmna −/− MEFs may harness other mechanisms to maintain normal heterochromatin and lamina-chromatin association and function as they exhibit similarly abundant and conspicuous heterochromatin foci as in WT MEFs, whereas differentiating Lmna −/− ESCs fail to organize heterochromatin ( Fig. 5e,f ). Taken together, these results suggest that LMNA affects chromatin plasticity during ESC early differentiation, restricting chromatin protein dynamics exclusively in heterochromatin, and is required for normal heterochromatin organization during ESC differentiation. In the absence of LMNA, differentiating cells fail to restrict chromatin protein dynamics, fail to obtain normal nuclear conformation and heterochromatin organization and display altered differentiation propensity. DNA methylation does not affect H1 dynamics in ESCs Obtained from the developing embryo's inner cell mass, ESCs have relatively low DNA methylation levels on derivation and they subsequently acquire DNA methylation during culturing [37] . Therefore, we hypothesized that DNA methylation might influence chromatin protein dynamics. To determine whether global DNA methylation levels contribute to the hyperdynamic nature of chromatin proteins in ESCs, we treated ESCs stably expressing H1–GFP with the DNA demethylating agents 5-Azacytidine (5-Aza) and Zebularine (Zeb) ( Supplementary Fig. S6a ) for 5 days, and performed FRAP analyses. We determined global DNA methylation levels using the nearest-neighbour method. We found that DNA methylation was reduced by ~30% following either 5-Aza or Zeb treatment ( Supplementary Fig. S6b ). Despite the decrease in DNA methylation levels, H1–GFP dynamics showed no significant changes following the different treatments ( Fig. 7 ). 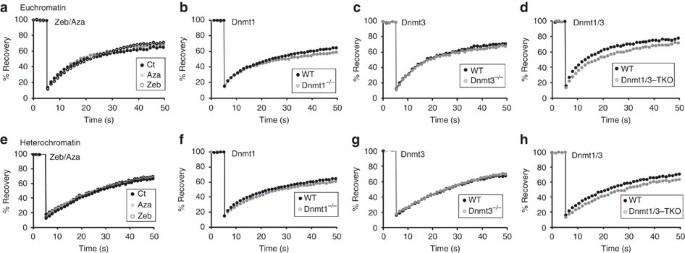Figure 7: DNA methylation does not affect H1 dynamics in ESCs. (a) H1e–GFP FRAP analysis in euchromatin of R1 ESCs, treated for 5 days with either 100 mM 5-Aza (grey) or 1 mM Zeb (empty) or untreated (Ct, black). (b) H1e–GFP FRAP analysis in euchromatin of Dnmt1 knockout ESCs (Dnmt1−/−, grey) compared with wild-type controls (WT, black). (c) H1e–GFP FRAP analysis in euchromatin of Dnmt3a/b double-knockout ESCs (Dnmt3−/−, grey) compared with wild-type controls (WT, black). (d) H1e–GFP FRAP analysis in euchromatin of Dnmt3a/b and Dnmt1 triple-knockout ESCs (Dnmt1/3-TKO, grey) compared with wild-type controls (WT, black). Changes are not significant (P=0.066, 2-tailedt-test). (e) H1e–GFP FRAP analysis in heterochromatin of R1 ESCs, treated for 5 days with either 100 mM 5-Aza (grey) or 1 mM Zeb (empty) or untreated (Ct, black). (f) H1e–GFP FRAP analysis in heterochromatin of Dnmt1 knockout ESCs (Dnmt1−/−, grey) compared with wild-type controls (WT, black). (g) H1e–GFP FRAP analysis in heterochromatin of Dnmt3a/b double-knockout ESCs (Dnmt3, grey) compared with wild-type controls (WT, black). (h) H1e–GFP FRAP analysis in heterochromatin of Dnmt3a/b and Dnmt1 triple-knockout ESCs (Dnmt1/3-TKO, grey) compared with wild-type controls (WT, black). Changes are not significant (P=0.07, 2-tailedt-test). Values are from at least 2 independent experiments, at least 20 cells each. Figure 7: DNA methylation does not affect H1 dynamics in ESCs. ( a ) H1e–GFP FRAP analysis in euchromatin of R1 ESCs, treated for 5 days with either 100 mM 5-Aza (grey) or 1 mM Zeb (empty) or untreated (Ct, black). ( b ) H1e–GFP FRAP analysis in euchromatin of Dnmt1 knockout ESCs (Dnmt1 −/− , grey) compared with wild-type controls (WT, black). ( c ) H1e–GFP FRAP analysis in euchromatin of Dnmt3a/b double-knockout ESCs (Dnmt3 −/− , grey) compared with wild-type controls (WT, black). ( d ) H1e–GFP FRAP analysis in euchromatin of Dnmt3a/b and Dnmt1 triple-knockout ESCs (Dnmt1/3-TKO, grey) compared with wild-type controls (WT, black). Changes are not significant ( P =0.066, 2-tailed t -test). ( e ) H1e–GFP FRAP analysis in heterochromatin of R1 ESCs, treated for 5 days with either 100 mM 5-Aza (grey) or 1 mM Zeb (empty) or untreated (Ct, black). ( f ) H1e–GFP FRAP analysis in heterochromatin of Dnmt1 knockout ESCs (Dnmt1 −/− , grey) compared with wild-type controls (WT, black). ( g ) H1e–GFP FRAP analysis in heterochromatin of Dnmt3a/b double-knockout ESCs (Dnmt3, grey) compared with wild-type controls (WT, black). ( h ) H1e–GFP FRAP analysis in heterochromatin of Dnmt3a/b and Dnmt1 triple-knockout ESCs (Dnmt1/3-TKO, grey) compared with wild-type controls (WT, black). Changes are not significant ( P =0.07, 2-tailed t -test). Values are from at least 2 independent experiments, at least 20 cells each. Full size image To reach lower levels of DNA methylation, we further analysed chromatin protein dynamics in ESCs lacking one or more DNA methyltransferase (DNMT) genes. We tested ESCs lacking the maintenance DNMT gene Dnmt1 [38] and ESCs lacking both de novo DNMT genes, Dnmt3a and Dnmt3b [39] . Nearest-neighbour analysis demonstrated that global DNA methylation levels were reduced by ~80% in Dnmt1 −/− cells and by more than 90% in Dnmt3 double knockout cells ( Supplementary Fig. S6b ). We note that this method gives a gross approximation, not absolute values, but our levels are in good agreement with previous reports [40] . FRAP analyses showed a very slight, statistically insignificant, increase in H1e–GFP dynamics in both Dnmt1 −/− ( Fig. 7b,f ) and Dnmt3a/3b −/− ( Fig. 7c,g ) ESCs tested. To exclude the possibility that DNMTs are functionally redundant with respect to chromatin dynamics, we further analysed ESCs lacking all three DNMT genes ( Dnmt1/3a/3b triple knockout (TKO)) [40] . In these Dnmt -TKO ESCs, we observed a slightly more pronounced increase in H1–GFP mobility, albeit not statistically significant ( Fig. 7d,h ). HP1–GFP and HMGN1–GFP both displayed similar kinetics between WT ESCs and the different mutants used ( Dnmt1 −/− , Dnmt3 −/− and Dnmt -TKO), as did H1–GFP ( Supplementary Fig. S7 ). As DNA methylation levels had very little effect on chromatin plasticity in undifferentiated ESCs, we searched for an effect during early differentiation. Although embryoid body (EB) formation kinetics were faster in Dnmt −/− ESCs than in WT cells, the double mutants failed to differentiate properly into NPCs ( Supplementary Fig. S8a–b ). We therefore induced differentiation, using RA, and analysed H1e–GFP dynamics after 24 and 48 h. Within 24 h of RA treatment, we observed no appreciable differences in H1e dynamics ( Supplementary Fig. S8c ) but within 48 h of RA treatment, we observed a notable restriction in H1e dynamics in Dnmt3 −/− ESCs when compared with WT ESCs ( Supplementary Fig. S8d ). This demonstrates that de novo DNA methylation is required during ESC differentiation, but suggests no involvement of DNA methylation in restriction of chromatin plasticity. Considering potential secondary effects on histone modifications in Dnmt knockout cells [41] , we examined histone acetylation and H3K9 methylation levels in Dnmt -TKO and WT cells, and found no significant differences ( Supplementary Fig. S8e ). These data indicate that with the exception of a small contribution to H1 dynamics, global levels of DNA methylation do not account for the altered dynamic nature of chromatin proteins in ESCs. Nucleosome spacing does not affect H1 dynamics in ESCs We then asked whether global changes in chromatin architecture, such as altered nucleosome spacing, would influence chromatin protein dynamics. We examined ESCs lacking three different H1 genes, H1c , H1d and H1e (H1 triple-knockout, H1-TKO) [42] , which have reduced chromatin repeat length and altered chromatin structure [43] . FRAP analysis demonstrated that the absence of these H1 variants did not affect H1–GFP dynamics ( Fig. 8 ). H1-TKO ESCs lack 50% of WT H1 levels [42] , so ectopically expressed H1–GFP might partially or fully restore H1 levels, rescue the H1 deficiency phenotype and thus obscure its effect on chromatin dynamics. We therefore compared HP1–GFP and HMGN1–GFP dynamics in H1-TKO cells versus WT ESCs, but neither protein had detectably different chromatin dynamics in these cells ( Fig. 8 ). These results suggest that reduced histone H1 levels in H1-TKO cells and the resulting altered chromatin structure do not affect chromatin protein dynamics and do not explain the observed differences in chromatin plasticity between ES and differentiating cells. 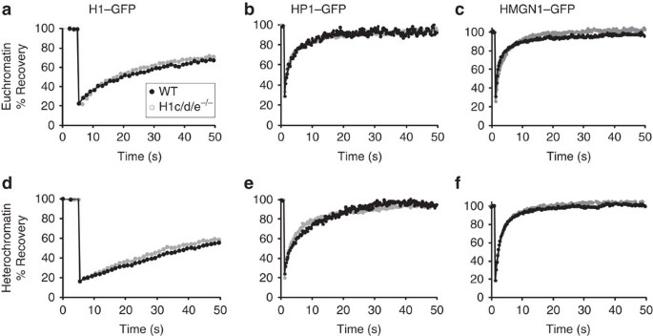Figure 8: Nucleosome spacing does not affect chromatin protein dynamics in ESCs. (a) H1e–GFP FRAP analysis in euchromatin of H1c/d/e triple-knockout ESCs (H1c/d/e−/−, grey) compared with wild-type controls (WT, black). (b) HP1–GFP FRAP analysis in euchromatin of H1c/d/e triple-knockout ESCs (grey) compared with wild-type controls (black). (c) HMGN1–GFP FRAP analysis in euchromatin of H1c/d/e triple-knockout ESCs (grey) compared with wild-type controls (black). (d) H1e–GFP FRAP analysis in heterochromatin of H1c/d/e triple-knockout ESCs (grey) compared with wild-type controls (black). (e) HP1–GFP FRAP analysis in heterochromatin of H1c/d/e triple-knockout ESCs (grey) compared with wild-type controls (black). (f) HMGN1–GFP FRAP analysis in heterochromatin of H1c/d/e triple-knockout ESCs (grey) compared with wild-type controls (black). No significant changes were observed for any of the tested proteins. Values are from at least 2 independent experiments, at least 20 cells each. Figure 8: Nucleosome spacing does not affect chromatin protein dynamics in ESCs. ( a ) H1e–GFP FRAP analysis in euchromatin of H1c/d/e triple-knockout ESCs (H1c/d/e −/− , grey) compared with wild-type controls (WT, black). ( b ) HP1–GFP FRAP analysis in euchromatin of H1c/d/e triple-knockout ESCs (grey) compared with wild-type controls (black). ( c ) HMGN1–GFP FRAP analysis in euchromatin of H1c/d/e triple-knockout ESCs (grey) compared with wild-type controls (black). ( d ) H1e–GFP FRAP analysis in heterochromatin of H1c/d/e triple-knockout ESCs (grey) compared with wild-type controls (black). ( e ) HP1–GFP FRAP analysis in heterochromatin of H1c/d/e triple-knockout ESCs (grey) compared with wild-type controls (black). ( f ) HMGN1–GFP FRAP analysis in heterochromatin of H1c/d/e triple-knockout ESCs (grey) compared with wild-type controls (black). No significant changes were observed for any of the tested proteins. Values are from at least 2 independent experiments, at least 20 cells each. Full size image Here we investigate mechanisms underlying hyperdynamic and plastic properties of chromatin observed in undifferentiated ESCs [7] . We find that histone hyper-acetylation enhances euchromatin dynamics in the undifferentiated state, H3K9 methylation affects both euchromatin and heterochromatin dynamics, and LMNA restricts heterochromatin dynamics in early differentiation. These observations are in agreement with the fact that ESCs are devoid of LMNA [3] and that ESC chromatin has relatively high levels of histone acetylation and relatively low levels of H3K9 methylation [6] , [7] , [13] , [14] , [16] , [18] , [19] . Importantly, these observations suggest a direct link between chromatin dynamics and ESC pluripotency. This notion is supported by the fact that increased histone acetylation caused by HDACi treatment, promotes and facilitates reprogramming of somatic cells into pluripotent cells and helps maintain ESCs in an undifferentiated state [44] , [45] . Moreover, re-expression of Oct4 during cell reprogramming has been shown to be inhibited by G9a-mediated H3K9 methylation [25] whereas the small molecule BIX-01294 (BIX), a G9a inhibitor, improves reprogramming efficiency of primary NPCs transduced with Oct4 and Klf4 alone to a level comparable to 4-factor transduction ( Oct4 , Klf4 , Sox2 and cMyc ) [46] . It thus seems that both histone modification pathways we identified here as important for chromatin plasticity are also important for pluripotency. Notwithstanding, Suv39h1/2 knockout ESCs displayed no phenotype regarding chromatin plasticity or differentiation when induced to differentiate into neurons. It is likely that Suv39h1/2 participate in alternate differentiation routes rather than neuronal. Supporting this notion is a recent report showing the specific targeting of Suv39h1 to bivalent genes on trophoblast lineage commitment [47] . LMNA presents an additional pathway to restrict chromatin plasticity. When ectopically expressed in WT ESCs, LMNA restricted heterochromatin dynamics, perhaps by its direct association with core histones [4] , [5] . Our results also raise the possibility of a connection between LMNA and pluripotency, differentiation, and reprogramming. One such potential link may be through restricting pervasive transcription during differentiation [48] , [49] . Tethering a genomic locus to the nuclear lamina in somatic cells, which was shown to restrict transcription [50] , was accompanied by LMNA accumulation at the tethered site. It would therefore be interesting to test whether LMNA expression restricts pervasive transcription in ESCs [6] , [51] . It is likely that additional mechanisms have a role in regulating chromatin plasticity in ESCs. ATP-dependent chromatin remodelling proteins, prevalent in undifferentiated ESCs [6] , are good candidates. Recently, Chd1 was shown to regulate pluripotency in ESCs [52] . We found that stable downregulation of Chd1 expression increased heterochromatin formation and reduced chromatin protein dynamics [52] , suggesting that Chd1 facilitates an open chromatin conformation in undifferentiated ESCs. It would be interesting to decipher the role(s) that other chromatin remodellers have in stem cell biology because accumulating evidence suggest they are highly important for the stem cell state [6] , [52] , [53] , [54] . Interestingly, we found that DNA methylation levels, although crucial for ESC differentiation, have very little role, if any, in regulating chromatin protein dynamics in ESCs. In another study [55] , a slight decrease in linker histone kinetics was observed in Dnmt3 −/− ESCs. Although these observations are in line with our measured kinetics in differentiating Dnmt3 −/− ESCs, we observed no differences in the undifferentiated state. This could be owing to differences in GFP-tag location, the nature of the linker histone used or differences between different ESC lines. Regardless, our studies indicate that DNA methylation is not a major factor responsible for the dynamic nature of chromatin proteins in ESCs. Perhaps more surprising is the fact that global chromatin structure had no apparent effect on chromatin protein dynamics in ESCs. ESCs lacking three linker histones displayed reduced local chromatin compaction and decreased global nucleosome spacing [42] but their chromatin dynamics remained unaltered. It is possible that local, not global, chromatin dynamics have been altered, but this cannot be detected using FRAP. To conclude, we provide mechanistic insight into our previous observations that chromatin proteins are hyperdynamic in ESCs. We demonstrate that reduced histone acetylation, increased H3K9 methylation and LMNA expression, all act to restrict chromatin plasticity during ESC differentiation. Thus, undifferentiated ESCs, which possess high levels of histone acetylation, relatively low levels of H3K9 methylation and no LMNA, are able to maintain a plastic chromatin state that supports pluripotency. Cells Mouse R1 and E14 ESCs were from ATCC; Dnmt1 −/− ESCs from R. Jaenisch (Cambridge, MA, USA); Dnmt3a/b −/− from E. Li (Cambridge, MA, USA), Dnmt1/3a/b −/− from M. Okano (Kobe), Suv39h1/2 −/− from T. Jenuwein (Freiburg); G9a −/− , GW1 (G9a addback), G44 (G9a mutant-addback) and TT2 (the parental strain of the 3 G9a derivatives) from Y. Shinkai (Kyoto). Pluripotent ESCs were grown on γ-irradiated or mitomycin-C-treated MEFs in DMEM, 10–15% ESC-grade FCS, 1 mM sodium pyruvate, 0.1 mM nonessential amino acids, 0.1 mM β-mercaptoethanol, and 1,000 U ml −1 LIF. LIF withdrawal differentiation was performed by separating ESCs from MEFs, plating them on gelatin-coated dishes and culturing in ES medium without LIF. RA-induced differentiation was performed in a similar way with the addition of 1 μM RA. For NPC differentiation, ESCs were separated from MEFs and grown in suspension on bacterial culture dishes without LIF for 4 days to allow for EB formation. EBs were replated on poly-l-ornithine/fibronectin (Sigma)-coated plates in DMEM/F12 medium supplemented with ITS (5 mg ml −1 insulin, 50 mg ml −1 transferrin, 30 nM selenium chloride) and fibronectin (5 mg ml −1 ) and grown for 2–6 days longer until NPC day 6–10, respectively. All cell culture media were supplemented with 2 mM glutamine, 100 U ml −1 penicillin, and 50 mg ml −1 streptomycin. All cell culture reagents were purchased from GIBCO-BRL (Invitrogen; Carlsbad, CA, USA). DNA transfections were performed with TransIt (Mirus) and Lipofectamine-2000, according to the manufacturer's instructions. For photobleaching experiments, cells were grown in 8-well μ-Slides (ibidi, Munich, Germany) or in chambered cover glasses (Lab-Tek; Rochester, NY, USA) or in glass-bottom culture dishes (MatTek; Ashland, MA, USA). 5-Aza, Zeb, TSA, VPA and AA were added to the cells at a final concentration of 0.5 μM, 200 μM, 50 nM, 0.5 mM and 50 μM, respectively. 5-Aza and Zeb were applied for 5 days. TSA and VPA were applied for 4 h, 16 h or 24 h. AA was applied for 1 h. Plasmids H1e–GFP, H1–GFP, HP1α–GFP, HMGN1–GFP and FLAG-HA–G9a fusion proteins have been previously described [7] , [15] , [17] , [22] , [56] , [57] . Stable R1 clones expressing GFP fusion proteins were generated by introducing the expression vectors via electroporation, selection for resistance to G418, followed by identification of expressing clones by direct observation under epifluorescence. For mouse Lmna ( mLmna ) cloning, total RNA was extracted from MEFs using the RNeasy Mini Kit (Qiagene) and complementary DNA was prepared using an RTase kit (Applied Biosystems). The mLMNA coding sequence was amplified by PCR with the following DNA oligos:5′-cgatctcgaggaatggagaccccgtcacagcg-3′; 5′-cgatggatccttacatgatgctgcagttctggg-3′ (Syntezza Bioscience, Israel). Products were separated in agarose gels and ligated into the T-Easy Vector system (Promega). The mLMNA coding sequence was inserted into the pmCherry-C2 vector (Clontech), using EcoRI, and orientation was verified by sequencing. To create a WT tag-less mLamin A expression vector, mCherry was excised with AgeI and BglII and the mLmna -containing vector was treated with Klenow and re-ligated. Antibodies and immunofluorescence The following antibodies were used at the corresponding concentrations: Nestin, 1:100 whole serum antibody (rabbit polyclonal), kindly provided by R. McKay (National Institutes of Health, Bethesda, MD, USA); LMNA, 2 μg ml −1 (rabbit polyclonal, sc-20680: Santa Cruz Biotechnologies, Santa Cruz, CA, USA); TUJ1, 1:200 ascites fluid (mouse monoclonal, MAB1637:Millipore); Oct4, 1 μg ml −1 (N19 goat polyclonal, sc-8628: Santa Cruz); Nanog, 10 μg ml −1 (Goat polyclonal, AF2729: R&D systems); HP1α1:750 ascites fluid (Mouse monoclonal, 2HP-1H5-As: Euromedex); H3K9me3, immunofluorescence (IF) 1:100, WB 1:1,000 serum antibody (Rabbit polyclonal), kindly provided by T. Jenuwein; H3Ac, 1 μg ml −1 (Rabbit polyclonal, 06-599: Upstate). Detection for WB was with anti-rabbit or anti-mouse antibodies conjugated to HRP (Rockland) and for IF with anti-rabbit, anti-mouse or anti-goat antibodies conjugated to Alexa488 or Alexa568 (Molecular Probes, Carlsbad, CA, USA), Cy3 or FITC (Jackson ImmunoResearch, West Grove, PA, USA). For IF, cells, grown either in 8-well μ-Slides (ibidi, Munich, Germany) on cover-slips, were fixed in 4% paraformaldehyde (15 min, room temp. ), washed 3 times in PBS (5 min, room temp), permeabilized with 0.5% Triton X-100 in PBS (5 min, room temp.) and incubated with the primary antibodies (1 h, room temp. or 4 °C overnight). Cells were then washed 3 times in PBS (5 min, room temp. ), incubated with secondary antibodies (1 h, room temp. ), washed again in PBS (5 min, room temp. ), DAPI stained (5 min, room temp. ), washed again in PBS (5 min, room temp.) and mounted on a microscope slide with anti-fade (Dako, Glostrup, Denmark). Microscopy and photobleaching Imaging was done as described [7] or using a Revolution spinning disk (CSUX, Yokogawa) imaging system (Andor, UK) with solid state lasers 405, 488, 561 and 640 nm (50 mW each) mounted on an Olympus IX81 fully automated microscope equipped with an automated stage, autofocus device (Z-drift compensation) and an environmental chamber (LIS, Switzerland) controlling oxygen, humidity, CO 2 and temperature. FRAP was done using a specialized FRAPPA module (Andor, UK) at 50–100% laser intensity as described [58] . Bleaching was confined to square areas of 15×15 pixels in MEFs and 12×12 pixels in ESCs and NPCs using a ×60 oil lens with a numerical aperture of 1.4. We used an EMCCD iXon+ camera (Andor, UK) with a window size of 512×512 pixels. When separately analysing euchromatin and heterochromatin, bleach areas were discretely positioned away from GFP-positive foci or directly on them, respectively. All FRAP analyses were performed on 15–30 cells from at least 2 independent experiments. Data analyses were as described [7] . Heterochromatin foci quantification was performed by manually counting DAPI dense foci that co-localize with HP1α and H3K9me3 immunostaining. This method was verified semi-automatically with ImageJ threshold analysis. Teratoma formation Ten million cells suspended in 35 μl ESC medium and 15 μl MatrigelTM (BD Biosciences) were injected subcutaneously into the dorsal flank of SCID mice (C.B-17/lcrHsd-SCID-bg). Three weeks after the injection, mice were killed and teratomas were surgically dissected. Samples were weighed, fixed in PBS containing 4% paraformaldehyde, embedded in paraffin and sliced into 7 μm-thin sections. Sections were stained with haematoxylin and eosin. The joint ethics committee (IACUC) of the Hebrew University and Hadassah Medical Center approved the study protocol for animal welfare. The Hebrew University is an AAALAC International accredited institute. All animal experiments were conducted in accordance with the Hebrew University's animal committee, ethical approval # IACUC:NS-09-11616-4. Nearest-neighbour analysis DNA methylation levels were determined using MboI digestion and end labelling as described in detail [59] . Statistical analyses Two-tailed Student's t -test was performed to compare the kinetics of the different FRAP curves. t -test was used to adhere to our previous analyses to allow comparisons [7] . We note that t -test in this regard is a conservative test and that other statistical tests (for example, Fisher's Omnibus), which take into account entire graphs may result in lower P -values. Graphs were compared at time t =40 s, and P -values were calculated on these comparable time points, as described [56] . How to cite this article: Melcer, S. et al . Histone modifications and lamin A regulate chromatin protein dynamics in early embryonic stem cell differentiation. Nat. Commun. 3:910 doi: 10.1038/ncomms1915 (2012).